Detection of microwave phase variation in nanometre-scale magnetic heterostructures The internal phase profile of electromagnetic radiation determines many functional properties of metal, oxide or semiconductor heterostructures. In magnetic heterostructures, emerging spin electronic phenomena depend strongly upon the phase profile of the magnetic field at gigahertz frequencies. Here we demonstrate nanometre-scale, layer-resolved detection of electromagnetic phase through the radio frequency magnetic field in magnetic heterostructures. Time-resolved X-ray magnetic circular dichroism reveals the local phase of the radio frequency magnetic field acting on individual magnetizations through the susceptibility as . An unexpectedly large phase variation, ~40°, is detected across spin-valve trilayers driven at 3 GHz. The results have implications for the identification of novel effects in spintronics and suggest general possibilities for electromagnetic-phase profile measurement in heterostructures. Many functional properties of heterostructures require a known phase relationship between electromagnetic (EM) fields throughout the structure. Lasing [1] , [2] , [3] , superconducting microwave properties [4] , [5] , negative refraction [6] , [7] and stimulated phonon emission (‘sasing’) [8] , [9] all require some degree of coherence in the EM phases across layers. Phase-sensitive electric fields have been measured for short light pulses in ionized gases [10] ; interferometric (wave mixing) techniques have been used to resolve the complex polarization of near band-edge absorption in single semiconductor quantum wells or thick films [11] . Nevertheless, these techniques have not been and perhaps cannot easily be applied to localize the phase of EM radiation in heterogeneous media. Layer- and interface-specific optical measurements, such as optical second harmonic generation [12] and photoluminescence [13] , have been limited to measurements of intensity ( | E | 2 ), losing information on the phase. Just as complex polarization can be used to investigate the complex electric field through dielectric susceptibility , magnetization can be used as a probe of complex magnetic fields through the magnetic susceptibility . Measurement of the complex radio frequency (rf) magnetic field profile is essential for interpretation of GHz phenomena in ferromagnetic heterostructures [14] , [15] , [16] , [17] . Asymmetric ferromagnetic resonance (FMR) lineshapes, which mix real and imaginary susceptibilities as have been interpreted in terms of imaginary effective field terms in the Landau-Lifshitz Gilbert (LLG) equation, attributed to novel spin transport mechanisms in heterostructures [15] , [16] , [17] . These interpretations typically rely on the assumption that there is no variation in the phase of reaching different ferromagnetic layers in a heterostructure. The use of ‘ultrathin’ ferromagnetic (F or FM) and normal-metal (N) films, much thinner than the metal skin depths δ as t F,N << δ , is widely believed to make propagation effects negligible, creating a constant, real-valued magnetic field profile H rf ( z ) =H 0 . Recent analysis has called this assumption into question [18] . In this article, we resolve the rf signal phase to 15 nm layers in a F 1 /N/F 2 heterostructure, demonstrating phase resolution of EM radiation inside a layered system. Time-resolved X-ray magnetic circular dichroism (TR-XMCD) provides a phase- and layer-specific measurement of magnetization M for structures excited near FMR. Based on for known of a single ferromagnetic layer, we determine the depth-dependent magnetic field . Even for thin N layers, for which k N t N <0.01, we find that the rf phase reaching ferromagnetic films F 1 , F 2 differs by as much as ~0.7 rad (40°). Comparison with a classical transfer-matrix model shows that moderate conductivity loss in the substrate, present in typical device structures, is enough to generate the observed layer-dependent phase. Insulating substrates, not treated in the experiment, are not expected to show comparable effects. Experimental We present data on three heterostructures deposited by ultrahigh vacuum sputtering. Two F 1 /N/F 2 trilayers were deposited as F 1 (15)/Cu(10)/F 2 (15 nm), with F 1 on the bottom, closer to the substrate, and F 2 on the top, closer to the rf source. In the first sample (‘Py/Cu/CoFeB’) F 1 =Ni 81 Fe 19 , F 2 =Co 60 Fe 20 B 20 . In the second sample (‘CoFeB/Cu/Py’), the deposition order was reversed: F 1 =Co 60 Fe 20 B 20 , F 2 =Ni 81 Fe 19 . Reversal of deposition order reverses any rf propagation delay experienced by a given layer. A third multilayer sample was deposited as a control, with a directly exchange coupled [Ni 81 Fe 19 (5 nm)/Co 60 Fe 20 B 20 (5 nm)] × 5 multilayer substituted for the trilayer. For this sample, we expect all F layers, strongly coupled through direct exchange, to precess in phase. TR-XMCD measurements were performed at Beamline 4-ID-C of the Advanced Photon Source, Argonne IL. XMCD enables measurement of element-specific magnetic moments through the circular dichroism of absorption at transition metal L 2,3 edges [21] , taking the projection of moments along the beam helicity direction σ ph as M ·σ ph . For elements which are not common between layers in a heterostructure, true for Ni and Co here, XMCD is a probe of layer-specific magnetization, able to characterize buried layers as pictured in Fig. 1a . TR-XMCD adds temporal resolution as a rf-pump/synchrotron-probe measurement of magnetization dynamics, taking advantage of the <50 ps full width at half maximum (FWHM) bunch length of the synchrotron. For continuous-wave-rf magnetic field excitation delivered through a coplanar waveguide (CPW), synchronous with the photon bunch clock, we determine the layer-specific phase and amplitude response of the magnetization as See Arena et al. [20] and the Methods section for details on instrumentation and sample mounting. 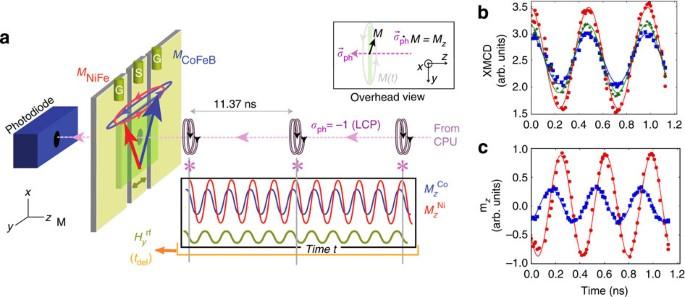Figure 1: Experimental method. (a) Illustration of the TR-XMCD technique. Stroboscopic X-rays, flashing at 40 ps, capture the precessional dynamics of individual magnetic layers in a heterostructure, through the Ni and Co circular dichroism signals at 854 and 779 eV, respectively, under continuous excitation at ~3 GHz. Variable delay time for rf excitation maps the temporal dependence (t=−tdel). (b) Dynamics in a [Ni81Fe19/Co60Fe20B20] × 5 multilayer, showing negligible phase difference between Ni81Fe19(Py) and Co60Fe20B20(CoFeB) layers. Red circles: Ni, Blue squares: Co, Green stars: Fe. Solid lines are sinusoidal fits. (c) Py(15 nm)/Cu(10 nm)/CoFeB(15 nm) sample, showing the bottom Py precession lagging, with higher phaseas, that of the top CoFeB layer:Py−Co>0. Magnetization precession amplitudefor Py is estimated ~10−3rad.; see Methods. arb. units, arbitrary unit. CPU, circularly polarizing undulator; LCP, left circurlarly polarized. Figure 1: Experimental method. ( a ) Illustration of the TR-XMCD technique. Stroboscopic X-rays, flashing at 40 ps, capture the precessional dynamics of individual magnetic layers in a heterostructure, through the Ni and Co circular dichroism signals at 854 and 779 eV, respectively, under continuous excitation at ~3 GHz. Variable delay time for rf excitation maps the temporal dependence ( t =− t del ). ( b ) Dynamics in a [Ni 81 Fe 19 /Co 60 Fe 20 B 20 ] × 5 multilayer, showing negligible phase difference between Ni 81 Fe 19 (Py) and Co 60 Fe 20 B 20 (CoFeB) layers. Red circles: Ni, Blue squares: Co, Green stars: Fe. Solid lines are sinusoidal fits. ( c ) Py(15 nm)/Cu(10 nm)/CoFeB(15 nm) sample, showing the bottom Py precession lagging, with higher phase as , that of the top CoFeB layer: Py − Co >0. Magnetization precession amplitude for Py is estimated ~10 −3 rad. ; see Methods. arb. units, arbitrary unit. CPU, circularly polarizing undulator; LCP, left circurlarly polarized. Full size image In the measurements presented, unlike those in Arena et al. [20] , we record only the (smaller) XMCD signal due to out-of-plane magnetization M z by measuring with incident X-rays (and helicity σ ph ) normal to the xy film plane, as pictured in Fig. 1a , inset . Normal incidence measurements exclude effects of ellipticity (differing ratio) on the phase of the TR-XMCD signal; see Methods. In Fig. 1b , we show validation and an estimate of uncertainty for the measurement of magnetization phase. In the [Ni 81 Fe 19 (5 nm)/Co 60 Fe 20 B 20 (5 nm)] × 5 multilayer sample, because the thicknesses are close to the exchange lengths ( δ ex ~5 nm) (ref. 22 ) and FMR properties are not very different for the layers, we expect mostly in-phase precession. In-phase precession is verified here to a resolution of 0.02 rad (6 ps). To calibrate the XMCD scale, we assume that the film-normal magnetization component m z is the same across interfaces during precession, inferring a Ni:Co XMCD signal ratio of 2:1 for equal m z = M z / M s . This relative calibration has been applied to the data presented in Figs 1c , 2 and 3a . 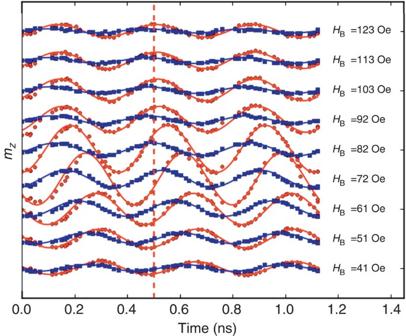Figure 2: Magnetic field bias dependence of layer-specific precession. TR-XMCD data, continuously driven precession at 2.694 GHz, for substrate/Py(15)/Cu(10)/CoFeB(15 nm)(top) trilayer sample. Variable magnetic field biasHBas indicated; data are offset for clarity. Blue squares: Co XMCD. Red circles: Ni XMCD. Lines: cosine fits with variable phaseand amplitude. Figure 2: Magnetic field bias dependence of layer-specific precession. TR-XMCD data, continuously driven precession at 2.694 GHz, for substrate/Py(15)/Cu(10)/CoFeB(15 nm)(top) trilayer sample. Variable magnetic field bias H B as indicated; data are offset for clarity. Blue squares: Co XMCD. Red circles: Ni XMCD. Lines: cosine fits with variable phase and amplitude . 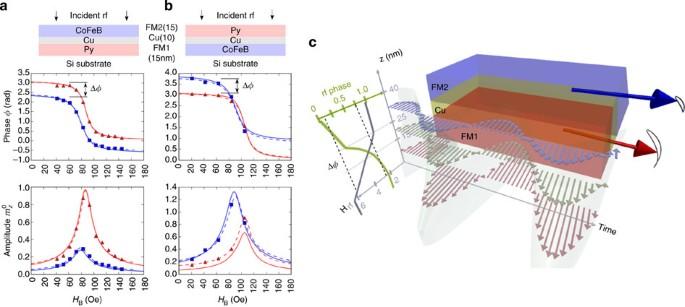Figure 3:Phase and amplitude of magnetization precession in the two layers. (a) Experimental magnetization phaseand amplitudefor substrate/Py(15)/Cu(10)/CoFeB(15 nm)(top) heterostructure, driven at 2.694 GHz, after sinusoidal fits inFig. 2, (b) for reversed-order substrate/CoFeB(15)/Cu(10)/Py(15 nm)(top) heterostructure, driven at 2.961 GHz (fits not shown), indicating phase offset Δ. Red: Ni (Py) resonance, blue: Co (CoFeB) resonance. Dashed lines: single-domain LLG fit, parameters after Ghoshet al.24(c) Calculated rf magnetic fieldphase profile(z) from transfer-matrix model, indicating phase offset Δ(green line, projected on left of Figure.) Field amplitude (Hrf, grey line) is normalized to the incident wave fieldHi; magnetization motion is indicated (not to scale). Solid lines ina,b: magnetization response calculated self-consistently from fields as shown inc. See text for details. Full size image Figure 3: Phase and amplitude of magnetization precession in the two layers . ( a ) Experimental magnetization phase and amplitude for substrate/Py(15)/Cu(10)/CoFeB(15 nm)(top) heterostructure, driven at 2.694 GHz, after sinusoidal fits in Fig. 2 , ( b ) for reversed-order substrate/CoFeB(15)/Cu(10)/Py(15 nm)(top) heterostructure, driven at 2.961 GHz (fits not shown), indicating phase offset Δ . Red: Ni (Py) resonance, blue: Co (CoFeB) resonance. Dashed lines: single-domain LLG fit, parameters after Ghosh et al. [24] ( c ) Calculated rf magnetic field phase profile ( z ) from transfer-matrix model, indicating phase offset Δ (green line, projected on left of Figure.) Field amplitude ( H rf , grey line) is normalized to the incident wave field H i ; magnetization motion is indicated (not to scale). Solid lines in a , b : magnetization response calculated self-consistently from fields as shown in c . See text for details. Full size image Layer-dependent magnetization dynamics for the Py/Cu/CoFeB sample, measured at 2.694 GHz, are shown in Fig. 1c . The precession of the Ni 81 Fe 19 (Py) layer (at the bottom of the trilayer, closer to the substrate) is shown to lag the precession of the Co 60 Fe 20 B 20 (CoFeB) layer (on the top, closer to the rf source). Taking the temporal dependence as with =+| k | z for a single propagating wave incident from the CPW, we see that the magnetization phase lag for the Py layer, further away from the rf source, is greater than that for the CoFeB layer, closer to the rf source. Additionally, the precessional amplitude for the Py layer is larger, roughly twice that of the CoFeB layer. Figure 2 shows the layer-resolved dynamics as a function of applied magnetic field H B . The bottom layer lags the top for all fields swept across resonance. The sweep goes from high field (driving frequency less than the resonant frequency, ω < ω 0 ) to resonance, with a maximum amplitude response, to low field ( ω > ω 0 ). In the downward field sweep, the phase (lag) of each layer advances by ~ π , as expected, each maintaining an offset with respect to the other. TR-XMCD data Extracted values of the layer-dependent magnetization phase and amplitude as a function of applied field H B , are shown in Fig. 3a . The variation of phase and amplitude, fitted according to the single-domain model in Chan et al. [23] with layer-specific parameters constrained from Ghosh et al. [24] , is shown in dashed lines. There is a rigid positive offset in precessional phase lag Δ = Py − CoFeB ~0.7 rad, and roughly twice the precessional amplitude for the bottom Py layer compared with that of the top CoFeB layer. We compare the behaviour of Py(15 nm)/Cu(10 nm)/CoFeB(15 nm) with that of a reversed deposition order CoFeB(15 nm)/Cu(10 nm)/Py(15 nm) structure in Fig. 3b . The roles of the two layers reverse: the bottom CoFeB layer is now phase-lagged compared with the top Py layer, as Δ = Py − CoFeB =−0.62 rad, and its precessional amplitude is increased, as . In this sample, we have measured TR-XMCD delay scans at five field values on the low-field side of resonance, compared with eleven field values spanning resonance for the Py/Cu/CoFeB sample in 3a. The rf field amplitudes in CoFeB/Cu/Py are thus determined with lower precision than in Py/Cu/CoFeB, reflected in the somewhat poorer fit to the model. We fitted a 5 Oe shift in resonance position for the CoFeB layer using a reduced surface anisotropy for the CoFeB/Cu interface; see Methods. Again, however, the bottom ferromagnetic layer, further away from the rf source and closer to the substrate, has both a higher phase lag and a higher precessional amplitude, by comparable magnitudes. The phase offset of rf magnetization response, primarily dependent upon depth z in the heterostructure, is most plausibly interpreted as an offset in the phase ( z ) of the driving field, . Similarly, the depth-dependent amplitude of the magnetization response suggests a depth-dependent rf field amplitude | H rf ( z )|. Both features are reproduced through EM simulation of the rf field profile, illustrated in Fig. 3c . The rf field profile, showing both phase ( z ) (green, top axis) and amplitude H rf ( z ) (grey, bottom axis), is projected to the left grid, as calculated for an applied field H B above the FMR fields for the two layers. Time-dependent rf magnetic fields at the midpoint of each layer, FM1(15 nm), Cu(10 nm), FM2(15 nm), are illustrated with red, yellow and blue arrows, respectively; elliptical magnetization motion is indicated, exaggerated in scale by two orders of magnitude for visibility. Calculations at fields below or between the layer resonances differ only slightly, by <15% in amplitude or phase. The magnetization response calculated self-consistently with the field profile shown in Fig. 3c is shown with solid lines in Fig. 3a,b . Good agreement is found: the simulation reproduces the salient rigid phase offset Δ and larger rf magnetic field amplitude nearer the substrate. The physical content of the simulations consists solely of Maxwell's equations for the conductors and the LLG equation for the ferromagnets, as outlined in classic work by Ament and Rado [25] . The layer-specific magnetization response is interpreted as a local measurement of complex, thickness-averaged magnetic fields in the layers. In the experiment, the layer magnetizations respond to time-dependent effective magnetic fields, not simply the rf auxillary fields sourced by the waveguides. Known sources of time-dependent effective fields include interlayer coupling: either magnetostatic/Neel, or dynamical/spin pumping [26] . Neither type of coupling will reproduce the phase offset observed and coupling has been neglected in the simulation. For effective fields from coupling alone, the influence on dynamics of layer i will be maximized near the FMR of layer j and become negligible at much higher or lower fields. While we cannot exclude the possibility that the phase offset arises in part from yet-unidentified terms to the LLG, propagation effects alone provide a sufficient and plausible interpretation of the results. Conductivity of the moderately doped Si substrate, supplied as a support for the membrane used in the experiment, has the most important role in generating the inhomogeneous fields and phase offset Δ , according to the simulation. The simulation (see Methods) shows that maintaining F, N and substrate layers much thinner than the skin depth, t i << δ 0 , does not ensure a homogeneous rf magnetic field through the film thickness, consistent with the results presented here. It is not clear to what extent the measured Δ ~0.6–0.7 rad is typical for spin-valve-type structures at frequencies near 3 GHz. We may comment that we have observed similar phase offsets 0.4<Δ <1.0 rad, never less, in a larger and less well-controlled set of spin-valve samples than those presented here. These structures have had thinner F layers (to 5 nm), thicker Cu layers (to 20 nm), different compositions of Co-rich layers, membrane supports used from two different manufacturers, film depositions carried out in three separate systems by three separate groups, and rf frequencies varying from 1.8 to 4.1 GHz. Nevertheless, our simulations predict (see Methods), though our experiments have not tested, that an appreciable phase offset, up to π , would be expected for a specific range of substrate resistivity, amounting to one or two decades, for a given substrate thickness. Only a negligible phase offset is predicted for an insulating, lossless substrate. The experimental results demonstrate that time-resolved, core-level X-ray spectroscopy can be used as a layer-specific, phase-resolved probe of EM radiation in a nanometre-scale heterostructure. We comment finally on perspectives of the technique. The full range of magnetoelectronic heterostructures, including magnetic tunnel junction stacks [27] and layers down to several nanometre thicknesses, are accessible at sheet level. Phase-resolved fields might also be probed with layer specificity in sub-micron patterned structures, using analogous focused X-ray techniques such as scanning transmission X-ray microscopy, applied recently to the study of smaller-angle precessional dynamics [28] . Finally, outside the domain of thin-film magnetism, depth-dependent -fields might be probed in dielectric or ferroelectric heterostructures using X-ray linear dichroism measurements of layer-specific polarization order [29] , particularly as novel light sources begin to probe THz and higher frequencies. Sample fabrication and mounting All layers were deposited on the flat side of Si 3 N 4 membrane windows, seeded by Ta(5 nm)/Cu(3 nm), and capped with Al(3 nm) to protect the layers beneath from oxidation. The AlO x side is placed closest to the CPW centre conductor (rf source) during TR-XMCD measurement. The commercial Si 3 N 4 membranes used doped Si 200 μm thick frames, rated at 1–30 Ω·cm resistivity. The Si 3 N 4 membrane thickness, transparent to soft X-rays in transmission, is 100 nm. A small (100 μm) hole has been drilled in the CPW centre conductor where the membrane is mounted during measurement; see Arena et al. [20] , Fig. 1 . TR-XMCD measurement The measurements were carried out at fixed helicity σ ph from the APS-4-ID-C circularly polarizing undulator (see Fig. 1a ). Samples were aligned to normal incidence by minimizing the XMCD signal in field-swept measurements . The out-of-plane magnetization amplitude during precession was not calibrated directly. In prior measurements at comparable input powers, slightly lower frequencies (2.2 GHz), and with ~30° incidence from normal, we measured an in-plane precessional angle 0.8° (ref. 19 ), or . For improved signal recovery, here we use lock-in detection of the XMCD signal, synchronous with rf power modulation at 5 kHz, as in Arena et al. [20] Given the expected ellipticity η of the Py precession, , we estimate the Py precession (units of ~1 in Fig. 1c ) at 0.07°, or 1.2 × 10 −3 rad. Calculations The response of magnetization to incident rf fields has been calculated using a transfer-matrix approach, suggested in Chan et al. [23] Kostylev [30] has investigated freestanding, conductive ferromagnetic bilayers excited by a single-sided stripline. The calculations shown in Fig. 3 are summarized here briefly; details will be published separately. We assume plane-wave microwaves, linearly polarized with E parallel to static magnetization , incident normal to the ‘top’ film side only. For the incident wave, electric field , magnetic field ( E i = H i for free space propagation), and wavevector For the reflected wave, H r =− E r . In Fig. 3c , left ( H − z plane), H rf / H i = H rf / E i ~2 as E r / E i ~−1 for the highly reflective film stack. At the opposite side (not film side) of the substrate, we assume a single transmitted wave propagating away from the surface into free space ( E t = H t , E t / E i = t ), where t is the calculated (order 10 −3 or less) transmission coefficient t = E t / E i of the full heterostructure with substrate. The assumption of plane-wave rf radiation, incident from a single (conductor) side and decaying to near zero intensity on the opposite side, is compatible with microstrip excitation and an approximation to excitation by a CPW, as discussed in Kostylev [30] . Transfer matrices M i for layers i link E and H fields at the top ( z =0) and bottom ( z = d i ) surfaces, where the individual film is bounded by 0 ≤ z ≤ d i , as ( cgs units) where the given, single wavenumber k form for M i is valid for diamagnetic or paramagnetic (not ferromagnetic) layers. In this formula, and the propagation constant p = H / E = k / k 0 is given in terms of the free-space wavenumber k 0 = ω / c . For the normal-metal Cu layers, the wavenumber k is given by the skin depth δ 0 , k =( j +1)/ δ 0 , where σ is the material conductivity in s −1 . For the Si substrate, we include the full Drude form with frequency-dependent effective dielectric constant ε eff , , ε eff = ε r +4 πj σ 0 / ω (1− jωτ ) −1 . We took ε r =11.7 and τ =100 fs, after (higher-frequency, W-band) experimental investigation of doped Si microwave properties. Both these matrices M have been validated against experimental data from the literature. For the conductive ferromagnetic layer, the determination of the transfer matrix M i is more involved and not easily written in closed form. The Rado-Ament analysis [25] requires that the fields in the conductive ferromagnet satisfy both microwave screening through the susceptibility-reduced skin depth, and the in-plane susceptibility according to the LLG equation, where the normalized field, frequency, and (spin-wave) wavenumber units are given in terms of the magnetization, gyromagnetic ratio γ, and exchange length δ ex , as h = H /(4 πM s ), Ω= ω /( γ 4 πM s ), and K = kδ ex . Generally, the skin depth expression, Eq. 2, favors the buildup of shorter-wavelength spin waves in the ferromagnet and the LLG expression, Eq. 3, favors longer wavelengths near the (uniform-mode) FMR frequency, tending to reduce the susceptibility near resonance for finite k . The Gilbert damping is represented as α . Equating in Eqs 2 and 3 and substituting for h eff in terms of K 2 from Eq. 4 leads to a bicubic expression for wavenumber k . There are then three combined spin-wave/microwave modes, which can propagate in either direction (or form odd and even combinations) through the film thickness. Assuming that no boundary conditions are given, the six mode amplitudes, with the four top and bottom electric and magnetic fields E (0), H (0), E ( d ), H ( d ), as in Eq. 1, together pose ten unknowns. Four constraints are given by continuity of electric and magnetic fields at the top and bottom surfaces; four additional constraints are given by torques on magnetization due to surface anisotropies (here taken as zero). The foregoing gives a system of ten (10) linear, homogeneous equations in eight (8) unknowns. Using LU decomposition, we reduce the system to the M matrix form in Eq. 1, two equations in four unknowns. The full transfer matrix of the stack, relating the electric and magnetic fields at the far side of the substrate to those at the top surface of the film, is given by the reverse-order product of the individual layer transfer matrices, M = M N −1 M N −2 ... M 1 M 0 , where i =0 is the first layer adjacent to the CPW (top side) and layer i = N −1 is the substrate, in this case Si, with substrate thickness t s =200 μm. The far-side boundary condition is given by E / E i = H / E i = t , where t = E t / E i is the transmissivity of the full stack. For the calculations, we used the following parameters. The values of 4 πM s , γ =( g eff /2)2 π· 2.799 MHz/ Oe , and surface anisotropy K s (used in 4 πM s eff =4 πM s −2 K s / M s ) for the Py and CoFeB layers, deposited as Py/Cu/CoFeB, were constrained to the values given in Ghosh et al. [24] , in which the layers were deposited identically. For 15 nm layers, these values yield 4 πM s eff = 9.604 kG (10.81 kG) for Py (CoFeB) and g eff =2.09 (2.07). Variations in effective damping α are allowed in the simulation for best fit, obtained for α =0.0095 for Py and 0.0125 for CoFeB. For the CoFeB/Cu/Py structure, deposited with reverse order, the surface anisotropy for the CoFeB layer was taken to be roughly half that in the reversed configuration. Electrical resistivites are also important for the EM simulation. We have taken representative values, not fitted, for ferromagnetic metal layers: ρ =20 μΩ·cm for Py, ρ =100 μΩ·cm for (amorphous) CoFeB. For Cu, we take ρ =10–12 μΩ·cm; the lower bound of Cu resistivity was used for the CoFeB/Cu/Py structure, the upper bound for Py/Cu/CoFeB, possibly reflective of growth variation. Any influence of boundary scattering/resistivity size effect has been lumped into these parameters. The resistivity of the Si substrate was an important fit parameter; the phase offset is responsive to the substrate resistivity. This value was specified only as a range by the manufacturer of the X-ray transparent membrane, 1–30 Ω·cm; we have taken 0.1 Ω·cm, slightly out of the specified range, for a fit to the experimental data. The effects of the seed, cap, and nitride layers have been excluded from the simulation for simplicity; these were not found to make important differences. Simulated results for the phase offset Δ as a function of substrate resistivity ρ Si are shown in Fig. 4 . For fixed substrate thickness t S , the largest deviations of phase shift from 0 and π are found for two regions of resistivity: one narrow region at higher ρ Si and one broader region at low ρ Si . Note that as the substrate becomes perfectly insulating, the phase offset predicted by the simulation tends towards zero. 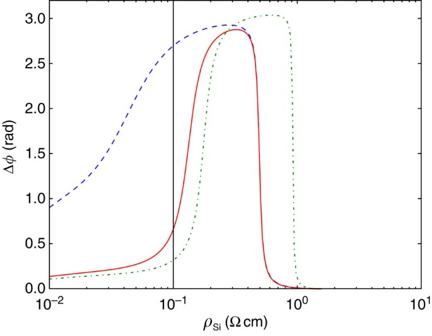Figure 4: Calculated phase offset. Calculated phase offset Δas a function of the Si substrate resistivityρSi. Solid line, with fittedρSi=0.1 Ω cm (vertical line), shows the configuration treated inFig. 3a; calculations for decreased Cu layer resistivity (ρCu=2.0 μΩ cm−1) and increased bottom Py layer resistivity (F1), (ρPy=40.0 μΩ cm−1) are shown in blue dashed and green dot-dashed lines, respectively. Figure 4: Calculated phase offset. Calculated phase offset Δ as a function of the Si substrate resistivity ρ Si . Solid line, with fitted ρ Si =0.1 Ω cm (vertical line), shows the configuration treated in Fig. 3a ; calculations for decreased Cu layer resistivity ( ρ Cu =2.0 μΩ cm −1 ) and increased bottom Py layer resistivity (F 1 ), ( ρ Py =40.0 μΩ cm −1 ) are shown in blue dashed and green dot-dashed lines, respectively. Full size image The conductive substrate (Si, or Si+other conductor) creates a magnetic field minimum at the incident surface for a specific ratio of substrate thickness t S to substrate skin depth δ 0 . Application of the transfer matrix, Eq. 1, predicts that is minimized for m 21 = m 22 (row-major) for unit transmission. Top-surface magnetic fields, nearer the rf source, are then minimized for substrate thickness t S ~ δ 0 ( k 0 δ 0 /2). Note that this magnetic field minimum does not occur for a substrate thickness equal to the skin depth, but rather for substrate thicknesses substantially thinner, in this case ~0.08 δ 0 , corresponding to ρ S =7.4 Ω·cm. Near this minimum, the phase of varies rapidly as a function of conductivity for fixed thickness t S . If a more conductive layer is introduced in contact with the substrate, on the same side as the rf source, the substrate resistivity ρ S for which the magnetic field is minimized shifts to lower values, for fixed t S . The high- ρ S region of large Δ occurs where the field at this surface is minimized, as the real part of H changes sign. Note that the position is sensitive to the bottom (F 1 ) layer resistivity, here Py, and shifts to lower ρ S for lower ρ Py . The phase variation in the top layer (F 2 ) is shifted to even lower values of ρ S , due to the larger thickness of conductive metal beneath it; we show that the breadth of this region is controlled by the Cu resistivity in the simulation, much broader for 2 μΩ·cm (near the lower bound for Cu) than for 15 μΩ·cm. The fields can thus become out of phase at different positions in the heterostructure, as found through the TR-XMCD measurements and reproduced in the simulations. How to cite this article: Bailey, W.E. et al. Detection of microwave phase variation in nanometre-scale magnetic heterostructures. Nat. Commun. 4:2025 doi: 10.1038/ncomms3025 (2013).